Enhanced proton transport in nanostructured polymer electrolyte/ionic liquid membranes under water-free conditions Proton exchange fuel cells (PEFCs) have the potential to provide power for a variety of applications ranging from electronic devices to transportation vehicles. A major challenge towards economically viable PEFCs is finding an electrolyte that is both durable and easily passes protons. In this article, we study novel anhydrous proton-conducting membranes, formed by incorporating ionic liquids into synthetic block co-polymer electrolytes, poly(styrenesulphonate- b -methylbutylene) (S n MB m ), as high-temperature PEFCs. The resulting membranes are transparent, flexible and thermally stable up to 180 °C. The increases in the sulphonation level of S n MB m co-polymers (proton supplier) and the concentration of the ionic liquid (proton mediator) produce an overall increase in conductivity. Morphology effects were studied by X-ray scattering and electron microscopy. Compared with membranes having discrete ionic domains (including Nafion 117), the nanostructured membranes revealed over an order of magnitude increase in conductivity with the highest conductivity of 0.045 S cm −1 obtained at 165 °C. Recently, ion-conducting polymers have attracted enormous attention for applications such as fuel cells, batteries and super capacitors [1] , [2] , [3] , [4] , [5] , [6] , [7] . Among the many kinds of ion-conducting polymers, proton-conducting polymers have been the subject of extensive study for their possible use in PEFCs, which offer the prospect of supplying clean energy for automotives. Significant efforts have been devoted to improving the transport properties of PEFCs so they can be operated at relatively lower temperatures below 90 °C [8] , [9] , [10] , [11] , [12] , [13] , [14] . However, the development of a commercial PEFC-powered vehicle that replaces a gasoline-powered vehicle still seems distant. One of the key challenges in advancing the technology lies in the long-term stability and durability of the system. Major issues are carbon monoxide (CO) poisoning of the platinum catalyst at the anode side, the complexity of heat and water management in polymer electrolyte membranes (PEMs), and the enhancement of reaction kinetics at both electrodes. Overcoming these issues may be simple if the operation performance of PEFCs is enhanced above 120 °C and a low-humidification condition is used. Above 120 °C, CO poisoning becomes negligible, and transport kinetics are significantly enhanced at higher temperatures [15] , [16] , [17] . Therefore, there is a growing need to develop a new system that can operate above 120 °C by replacing water with solvents that are non-volatile, have high boiling points and have high proton conductivities to alleviate the durability concerns. Ionic liquids are molten salts at room temperature, exhibiting non-volatility, thermal stability and negligible vapour pressures [18] . Excellent ionic conductivity up to the degradation temperature can open great possibilities regarding the high-temperature PEFC application [19] , [20] . Among various ILs, imidazolium-based ILs are the most widely studied, and poly(vinylidenefluoride-co-hexafluoropropylene) is a commonly used PEM material. However, as PVdF-HFP does not have protonic sites, the conductivities of the composite membranes generally depend on intrinsic properties, such as viscosity and conductivity, of the ILs. The reported conductivities range from 10 −4 to 10 −3 S cm −1 (refs [21] , [22] , [23] ). When Nafion, a current state-of-the-art PEM, is impregnated with different ILs, the reported anhydrous conductivity lies in the range of 0.001−0.1 S cm −1 at 100−200 °C [24] , [25] , [26] . Note that the conductivities of Nafion/IL systems are significantly dependent on variables such as the sample preparation temperature and casting solvent [27] , [28] , [29] . The reason for this ambiguity is not entirely clear as the morphology of Nafion remains unresolved. Based on the efforts to reduce the costs of membranes, the morphologies and proton conductivities of hydrocarbon-based PEM/IL composite systems with sulphonated poly(aryl ether ketone) (SPAEK) and poly(ethyl ether ketone) (SPEEK) have recently been investigated [26] , [29] . An ionic conductivity of ∼ 1×10 −2 S cm −1 is obtained at 180 °C when large amounts of ILs are incorporated. However, the conductivity is unsatisfactory when compared with the properties obtained with fully hydrated systems, and further improvements are needed. It should be noted here that SPAEK, SPEEK and Nafion have randomly organized ion-conducting channels with various length scales. Discrete domains of ion-conducting phases are inappropriate for charge transport, so introducing ordered ionic domains in the membranes is essential to attain improvement in the transport properties of PEFCs [30] , [31] , [32] , [33] , [34] . There are a few elegant studies on the ionic conductivity of polymerized ILs that explore the effect of the length of the spacers between the polymer backbone and the ionic moiety [17] , [33] , [34] . However, the reported ionic conductivities are low when compared with composite membranes due to the restricted motions of the ionic moiety. In this study, we were motivated to prepare novel anhydrous proton-conducting membranes by incorporating ILs into block co-polymer matrices. The system of interest consists of nearly monodisperse poly(styrenesulphonate- b -methylbutylene) co-polymers. In our system, −SO 3 H groups function as proton-active sites, and a greater amount of −SO 3 H groups can enhance conductivity, which can be achieved by synthetic controls. Our system shows spontaneous self-assembly on the ∼ 10 nm length scale, leading us to establish a synergetic way to obtain the maximum proton conductivity by adjusting the types of nanostructures, size of the ion-conducting channels, amount of incorporated IL and number of protonic sites in the matrix PEMs. Anhydrous proton transport in S n MB m /IL composite membranes The proton-conducting S n MB m /IL composite membranes were devised for elevated PEFC operating temperatures (above 120 °C). 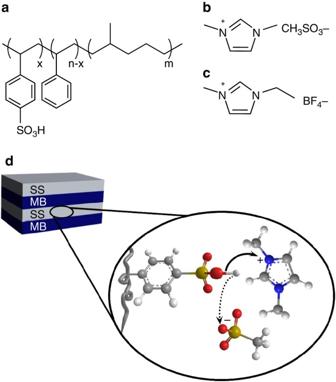Figure 1: Molecular structures and proposed proton hopping mechanism. (a) Poly(styrenesulphonate-b-methylbutylene) co-polymer (SnMBm), (b) 1,3-dimethylimidazolium methane sulphonate ([MMIm][MS]) and (c) 1-ethyl-3-methylimidazolium tetrafluoroborate ([EMIm][BF4]). (d) A schematic illustration showing the proposed proton hopping mechanism in SnMBm/[MMIm][MS] composite membranes. The protons transfer from –SO3H sites of SnMBmto MS anions of the ionic liquid are occurred by the conversion of hydrogen bond into covalent bond. The solid arrow and dashed arrow indicate the movement of electron and proton, respectively. The molecular structures of the S n MB m co-polymer, 1,3-dimethylimidazolium methane sulphonate ([MMIm][MS]) and 1-ethyl-3-methylimidazolium tetrafluoroborate ([EMIm][BF4]) are shown in Figure 1a–c respectively. The MS anion was chosen so as to contain sulphonate groups to ensure chemical similarity with styrenesulphonate (SS) chains. The direct comparison of [EMIm][BF4] and [MMIm][MS] allows the study of the effect of the chemical compatibility of pure ILs with S n MB m on the conductivity of composite membranes. The ionic conductivities of pure [EMIm][BF4] and [MMIm][MS] are qualitatively similar in the temperature window of our interest ( Table 1 ). Figure 1d illustrates the S n MB m nanodomains containing IL selectively within SS domains. The proposed proton conduction mechanism of our composite membranes is depicted in the enlarged circle for when [MMIm][MS] is used. The protons generated from –SO 3 H groups of SS chains associate with MS, and hopping and diffusion carry protons from one SO 3 − site to others along the SS domains. The ion transport mechanism of PEMs/[EMIm][BF4] is well described elsewhere [23] . Figure 1: Molecular structures and proposed proton hopping mechanism. ( a ) Poly(styrenesulphonate- b -methylbutylene) co-polymer (S n MB m ), ( b ) 1,3-dimethylimidazolium methane sulphonate ([MMIm][MS]) and ( c ) 1-ethyl-3-methylimidazolium tetrafluoroborate ([EMIm][BF4]). ( d ) A schematic illustration showing the proposed proton hopping mechanism in S n MB m /[MMIm][MS] composite membranes. The protons transfer from –SO 3 H sites of S n MB m to MS anions of the ionic liquid are occurred by the conversion of hydrogen bond into covalent bond. The solid arrow and dashed arrow indicate the movement of electron and proton, respectively. Full size image Table 1 Characteristics of block co-polymer electrolytes and ionic liquids used in this study. Full size table We first examined the temperature-dependent anhydrous proton conductivity by varying the number of proton-active sites provided by the polymer matrix (SL) and the number of proton mediators (IL concentration). 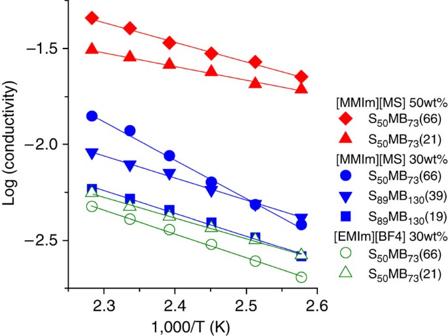Figure 2: Temperature-dependent in-plane conductivities of SnMBm/IL composite membranes. Conductivities of SnMBmmembranes with different molecular weights and sulphonation levels. The types of ionic liquids and the IL concentrations are indicated in the figure caption. The linear fits were obtained by Arrhenius plots. As plotted in Figure 2 , with an increase in the amount of absorbed IL and SL of S n MB m , the proton conductivity tends to increase. Higher temperatures increase the conductivity due to the enhanced charge transport, and the conductivity values reported in Figure 2 provide reproducible results without any change in sample colour or turbidity up to five heating/cooling cycles ranging between 25 and 165 °C. This suggests good thermal stability in this temperature regime. The activation energy ( E a ), obtained by Arrhenius plots, ranges between 14 and 35 kJ mol −1 . It is interesting to note here that, as clearly seen from Figure 2 , the incorporation of [EMIm][BF4] results in significantly lower conductivities than those achieved when using [MMIm][MS] at the same level of IL loading. The interfacial immiscibility between the hydrocarbon S n MB m and fluorinated anion is apparently attributed to the reduction of proton hopping along SS domains [24] . Figure 2: Temperature-dependent in-plane conductivities of S n MB m /IL composite membranes. Conductivities of S n MB m membranes with different molecular weights and sulphonation levels. The types of ionic liquids and the IL concentrations are indicated in the figure caption. The linear fits were obtained by Arrhenius plots. Full size image Morphology study of the composite membranes For brevity, we will only discuss representative data obtained from a subset of the samples listed in Table 1 . 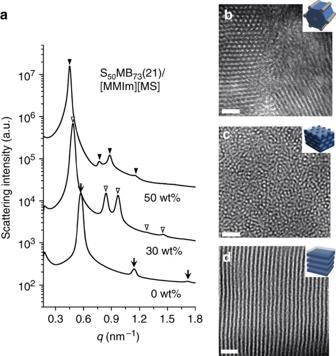Figure 3: Morphologies as a function of IL concentration. (a) SAXS profiles of S50MB73(21)/[MMIm][MS] composite membranes as a function of IL loadings at 150 °C. The arrows (↓) for 0 wt% IL, the inverted open triangles (▿) of 30 wt% IL and the inverted filled triangles (▾) of 50 wt% IL indicate Bragg peaks atq*, 2q*, 3q*; atq*,,,,; and atq*,,,, respectively. The scattering profiles are vertically offset for clarity. (b) Cross-sectional TEM images of 0 wt% IL, (c) 30 wt% IL and (d) 50 wt% IL show LAM-to-HPL-to-HEX phase transition structures on increasing IL loadings. The scale bars represent 50 nm. The schematic illustration of each nanostructure is shown in the figure as an inset box. The PSS domain was darkened by RuO4staining. Figure 3a shows small-angle X-ray scattering (SAXS) profiles obtained from S 50 MB 73 (21)/[MMIm][MS] by varying the amount of IL absorbed. Note that the SAXS profiles of all samples are independent of temperature up to 180 °C. When 30 wt% [MMIm][MS] is added to the lamellar forming S 50 MB 73 (21), the SAXS profile reveals a series of Bragg peaks ( ) at q *, , , , and , where q *=2 π / d 100 with d 100 =12.9 nm. A further increase in the IL loading to 50 wt% indicates the same ratio of Bragg peaks ( ) with d 100 =14.0 nm, indicative of hexagonally packed structures [35] . The q * value changes by 17% on loading with 30 wt% IL and further decreases by 27% with 50 wt% IL. This indicates the formation of larger domain sizes on the incorporation of IL due to the effective swelling of SS domains that occurs in the presence of [MMIm][MS]. Figure 3: Morphologies as a function of IL concentration. ( a ) SAXS profiles of S 50 MB 73 (21)/[MMIm][MS] composite membranes as a function of IL loadings at 150 °C. The arrows (↓) for 0 wt% IL, the inverted open triangles ( ▿ ) of 30 wt% IL and the inverted filled triangles ( ▾ ) of 50 wt% IL indicate Bragg peaks at q *, 2 q *, 3 q *; at q *, , , , ; and at q *, , , , respectively. The scattering profiles are vertically offset for clarity. ( b ) Cross-sectional TEM images of 0 wt% IL, ( c ) 30 wt% IL and ( d ) 50 wt% IL show LAM-to-HPL-to-HEX phase transition structures on increasing IL loadings. The scale bars represent 50 nm. The schematic illustration of each nanostructure is shown in the figure as an inset box. The PSS domain was darkened by RuO 4 staining. Full size image Qualitative differences exist in the SAXS profiles obtained with 30 wt% IL and 50 wt% IL loadings. Because the high-order reflections of hexagonally perforated lamellae (HPL and AB stacking) are identical to those of the hexagonal cylindrical phase (HEX), transmission electron microscopy (TEM) must be used to further illustrate the nature of obtained nanostructures. The TEM micrographs are shown in Figure 3b–d . Without IL, the TEM images indicate well-defined lamellar structures. The domain spacings of the composite membranes obtained from SAXS and TEM are identical. With 30 wt% IL, the TEM image ( Fig. 3c ) shows the presence of short lamellae with perforations and a hexagonal arrangement of the perforations, which leads to the conclusion that the structure is HPL. In contrast, Figure 3d clearly indicates the co-existence of [111] and [100] views of the HEX structure for the 50 wt% IL-containing sample. The nanostructures and swelling behaviour of S n MB m co-polymers are sensitive to the type of incorporated ILs. Contrary to the distinct swelling behaviour of S n MB m by incorporating [MMIm][MS], a fairly small change in domain size was detected for both S 89 MB 130 and S 50 MB 73 when [EMIm][BF4] was added. With 10 wt% of [EMIm][BF4] loading, a 5% increase in domain size was observed. However, on further increase in IL amounts, a gradual decrease in domain size was detected. At 50 wt% of [EMIm][BF4] loading, the domain size was almost identical to that of pure S n MB m ( Supplementary Fig. S2 ). This is undoubtedly due to the incompatibility between the PSS domains and [BF4] anions. Our study results resemble the phase behaviour of conventional block co-polymers/neutral solvent systems in which the decreased segregation results in decreased chain stretching normal to the interface [36] . Consequently, a large portion of the IL window studied is taken up by the same lamellar phase with the use of [EMIm][BF4] ( Supplementary Fig. S3 ). 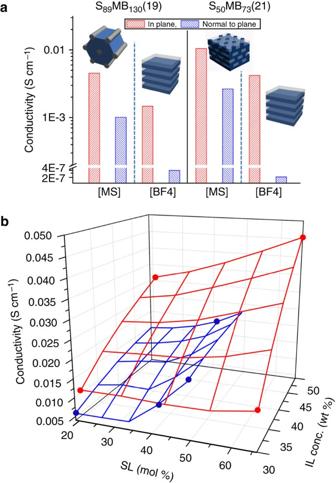Figure 4: Effects of IL type and molecular weight of SnMBmon conductivity. (a) The in-plane and normal-to-plane conductivities of S89MB130(19)/[MMIm][MS], S89MB130(19)/[EMIm][BF4], S50MB73(21)/[MMIm][MS] and S50MB73(21)/[EMIm][BF4] membranes at 30 wt% IL andT=150 °C. (b) The in-plane conductivity of SnMBm/[MMIm][MS] composite membranes obtained at 165 °C by varying the SL of SnMBmand the IL concentration. The red surface of the plot represents the in-plane conductivity of S50MB73/[MMIm][MS], and the blue plot the in-plane conductivity of S89MB130/[MMIm][MS]. Effects of IL type on conductivity To elucidate the effect of compatibility between ILs and PEMs (and the resulting different nanostructures) on conductivity, the anhydrous proton conductivities of S n MB m containing two ILs at a fixed loading of 30 wt% are plotted in Figure 4a . The samples were equilibrated at T =150 °C for 1 day before measurements. We first measured the in-plane conductivity ( σ ∥ ) and normal-to-plane conductivity ( σ ⊥ ) of HEX-forming S 89 MB 130 (19)/[MMIm][MS] and found σ ∥ =4.54 mS cm −1 and σ ⊥ =1.01 mS cm −1 ( σ ∥ / σ ⊥ =4.5). The lack of equality of σ ∥ and σ ⊥ is due to a coinciding of the current and voltage sensing paths as well as to the surface effects in the two-probe methods [37] , [38] . Figure 4: Effects of IL type and molecular weight of S n MB m on conductivity. ( a ) The in-plane and normal-to-plane conductivities of S 89 MB 130 (19)/[MMIm][MS], S 89 MB 130 (19)/[EMIm][BF4], S 50 MB 73 (21)/[MMIm][MS] and S 50 MB 73 (21)/[EMIm][BF4] membranes at 30 wt% IL and T =150 °C. ( b ) The in-plane conductivity of S n MB m /[MMIm][MS] composite membranes obtained at 165 °C by varying the SL of S n MB m and the IL concentration. The red surface of the plot represents the in-plane conductivity of S 50 MB 73 /[MMIm][MS], and the blue plot the in-plane conductivity of S 89 MB 130 /[MMIm][MS]. Full size image When the same amount of [EMIM][BF4] was added to the S 89 MB 130 (19), we saw a large reduction in σ ⊥ to 1.01×10 −4 mS cm −1 , and σ ∥ was approximately one third of that with [MMIm][MS]. This is because conductivity requires connectivity of microdomains across macroscopic length scales. In the lamellar forming S 89 MB 130 (19)/[EMIM][BF4], a non-random domain orientation occurs during the solution-casting process, and the alternating sequence of conducting domains and non-conducting domains significantly hinders proton conduction in the normal-to-plane direction. Qualitatively similar behaviour is observed for the low-molecular-weight S 50 MB 73 (21) sample. HPL-forming S 50 MB 73 (21)/[MMIm][MS] shows values of σ ∥ =10.49 mS cm −1 and σ ⊥ =2.66 mS cm −1 ( σ ∥ / σ ⊥ =3.9), whereas LAM-forming S 50 MB 73 (21)/[EMIM][BF4] results in σ ∥ =4.21 mS cm −1 and σ ⊥ =2.08×10 −4 mS cm −1 ( σ ∥ / σ ⊥ =2×10 4 ). The anhydrous σ ∥ of all S n MB m /[MMIm][MS] samples as a function of SL and IL concentration are plotted inside a cube in Figure 4b , obtained at 165 °C. All measurements were performed inside a glove box equipped with oxygen and moisture sensors, which reported values below 0.5 p.p.m. during the experiments. The red surface of the plot represents the σ ∥ of S 50 MB 73 /[MMIm][MS], and the blue plot surface located beneath represents that of S 89 MB 130 /[MMIm][MS]. The surfaces within the cube were obtained using a Renka–Cline gridding algorithm, which is part of the OriginPro 7.5 software package. As shown in Figure 4b , the increase in SL and IL concentrations produces an overall increase in conductivity, and the highest conductivity achieved for the S n MB m /[MMIm][MS] systems was 0.045 S cm −1 (45 mS cm −1 ) when 50 wt% [MMIm][MS] was incorporated into S 50 MB 73 (66). The low-molecular-weight S 50 MB 73 shows a twofold higher conductivity than the high–molecular-weight S 89 MB 130 . This is presumably because of the enhanced proton conduction by the low-viscosity ( η ) polymer matrix. The η of S 89 MB 130 (19) is expected to be roughly 1.3 times larger than that of S 50 MB 73 (21), estimated from the simple relationship [ η ] ∼ [ M ] ½ (ref. 39 ). A concrete interpretation of viscosity for charged polymers is complicated by several factors, including the sequence distribution of the ionic moiety and interactions between repeat units. The conductivity obtained with our synthetic S n MB m systems is orders of magnitude greater than the conductivity obtained with other systems reported [21] , [22] , [23] , [26] , [29] at the same temperature. An important phenomenon was observed in this study. When we carried out the same experimental protocol with the sulphonated S n homopolymers ( n =60 and 190), independent of the amount of absorbed IL, the samples flowed at temperatures higher than 100 °C (slightly above T g of sulphonated S n ). This is quite surprising because S n MB m co-polymers contain almost 50 vol% MB chains, and the mechanical strength of MB is very poor ( T g of MB chains is below 0 °C). This observation indicates that the self-assembly of S n MB m co-polymers into nanodomains provides enhanced mechanical strength at high temperatures. Note that all S n MB m /IL membranes reported here do not show order–disorder transitions at temperatures between 25 and 180 °C. We show temperature-dependent SAXS profiles from S 50 MB 73 (21)/[MMIm][MS] membranes in Supplementary Figure S4 . At a temperature of 95 °C, the σ ∥ values obtained with S 60 (32) and S 190 (33) doped with 30 wt% [MMIm][MS] loading were 0.13 and 0.78 mS cm −1 , respectively. With homemade liquid cells (two-probe configuration), we were able to measure the σ ⊥ of S 60 (32) and S 190 (33) as a function of IL concentration and temperature. Note that for the case of S 60 (32) and S 190 (33), the σ ∥ / σ ⊥ ratio was relatively small with a value of 1.4, presumably due to the vanished morphological effects. The higher IL concentrations gave higher conductivities, with values of 0.79 mS cm −1 (S 190 (33)/30 wt% IL), 1.0 mS cm −1 (S 60 (32)/30 wt% IL) and 3.4 mS cm −1 (S 60 (32)/50 wt% IL) at 150 °C, which are at least an order of magnitude smaller than that of S n MB m /[MMIm][MS]. Interestingly, the E a of the sulphonated S n homopolymer lies within 43–59 kJ mol −1 , which is twofold larger than that of S n MB m co-polymer systems. 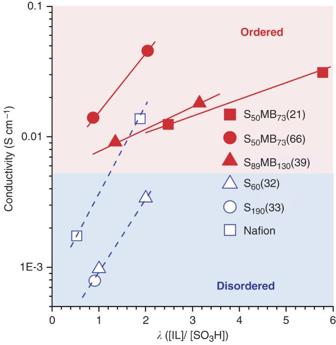Figure 5: Enhanced proton transport with nanostructured SnMBm/IL membranes. The in-plane conductivity of SnMBm/IL composite membranes and Nafion 117/IL as well as normal-to-plane conductivity of Sn/IL membranes as a function of the amount of absorbed IL per sulphonic acid group (λ) at 165 °C under anhydrous conditions. The amount of absorbed IL per sulphonic acid group ( λ ) was calculated and is shown in Figure 5 . This calculation estimates the effect of local ion concentrations on conductivity. The local concentration of cations/anions seems to be an important parameter for determining the efficiency of proton transport. For example, samples with higher SL (lower local concentrations of IL) have an increased probability of protonic site/cation/anion association; thus, the efficiency of net charge transport is improved. As summarized in Figure 5 , the conductivity obtained with our synthetic S n MB m /[MMIm][MS] system is fourfold enhanced compared to that of Nafion 117/[EMIm][BF4]. For the case of Nafion 117, we reported conductivity values obtained with [EMIm][BF4] rather than with [MMIm][MS] because the use of fluorinated [BF4] anions always gives higher conductivities for the entire temperature and IL concentration windows [23] , [24] . The effects of compatibilities of various ILs and polymer matrices on transport behaviour will be the subject of future studies. Figure 5: Enhanced proton transport with nanostructured S n MB m /IL membranes. The in-plane conductivity of S n MB m /IL composite membranes and Nafion 117/IL as well as normal-to-plane conductivity of S n /IL membranes as a function of the amount of absorbed IL per sulphonic acid group ( λ ) at 165 °C under anhydrous conditions. Full size image We conclude this article by highlighting the advantages of using nanostructured PEM. The conductivities obtained with nanostructured S n MB m /IL composite membranes are orders of magnitude higher than those with the S n /IL membranes lacking organization. If we assume that the conductivity of the hydrophobic phase is negligible, the maximum conductivity in PEM is given by σ max = σ h φ h , where σ h and φ h are the intrinsic conductivity and volume fraction of the conducting domains respectively. Our S n MB m possesses approximately 50 vol% conducting domain, and the simplest calculation gives a reduction in conductivity by half compared with S n , which is exactly the opposite of what we observed. This could be intimately related to the enhanced ion transport rate by creating a shortcut for charge transport, such as selective proton transport along the S n chains using imidazolium solvation groups (−SO 3 H sites) that are arranged into nanoscale domains. Synthesis of polymer electrolyte membranes S n MB m block co-polymers were synthesized by anionic polymerization of styrene (S) and isoprene (I) monomers followed by selective hydrogenation of isoprene to yield methylbutylene (MB) chains. The subscripts 'n' and 'm' represent the degree of polymerization for S and MB units, respectively. Styrene was purified by stirring over calcium hydride for 12 h, followed by vacuum distillation with n -butyl lithium for 6 h. Isoprene was treated with dibutyl magnesium for 3 h, followed by n -butyl lithium for 6 h. Cyclohexane was used as the polymerization solvent and was distilled from n -butyl lithium. Using sec -butyl lithium as an initiator, the styrene was polymerized for 4 h at 45 °C, followed by the addition of isoprene and polymerization for 4 h at the same temperature. The obtained polymers are S 89 I 130 and S 50 I 73 , which were characterized by gel permeation chromatography and by NMR (Bruker AVB-300) spectroscopy. The polydispersity indices of both polymers are less than 1.03. The saturation of SI co-polymers is performed in the presence of a homogeneous Ni-Al catalyst, using a 2 liter Parr batch reactor at 80 °C and 420 p.s.i. The Ni-Al catalyst was prepared by combining 50 ml of 0.1 M Nickel 2-ethylhexanoate in cyclohexane (Sigma-Aldrich) with 20 ml of 1.0 M triethylaluminum in heptanes (Sigma-Aldrich). After the reaction, the catalyst was removed by vigorously stirring the reaction mixture with 10% aqueous citric acid. The hydrogenated block co-polymers are referred to as S 89 MB 130 and S 50 MB 73 . The S chains of the S n MB m co-polymers were then partially sulphonated using procedures described as follows: 40 ml 1,2-dichloroethane and 1 g S n MB m were added to 100 ml three-neck flask equipped with a funnel and condenser. The mixture was heated to 40 °C under an N 2 blanket and stirred until the co-polymer was dissolved. Acetic sulphate was prepared by injecting 1.8 ml acetic anhydride and 5.4 ml dichloroethane into a sealed N 2 purged round-bottomed flask. The solution was cooled to 0 °C and 0.5 ml of 96% sulfuric acid was injected into the flask. The acetic sulphate was immediately transferred to the flask containing the S n MB m /dichloroethane mixture at 40 °C using a funnel. The reaction was terminated with 20 ml 2-propanol. Samples with different sulphonation level (SL) were prepared by controlling reaction time; SL=17±3 mol% with 0.25 h reaction, SL=37±4 mol% with 1 h reaction, SL=49±2 mol% with 4 h reaction and SL=63±3 mol% with 25 h reaction. Supplementary Figure S1 shows SL as a function of reaction time. The polymer in the reaction mixture was purified by dialysis against pure water using a cellulose dialysis membrane with a 3.5 kg mol −1 molecular weight cutoff (VWR) for 10 days. The polymer was then recovered by vacuum drying at 50 °C for 7 days. The molecular structure of resulting materials is shown in Figure 1a where SL of S n MB m was calculated by the equation given below: The SL value of the co-polymer is given in parentheses, i.e., S 89 MB 130 (39) contains 89 S chains and 130 MB chains where 39 mol% of S is sulphonated. The characteristics of S n MB m co-polymers used in this study are listed in Table 1 . Ionic liquids [MMIm][MS] (≥99% HPLC grade) and [EMIm][BF4] (≥98% HPLC grade) were purchased from Sigma-Aldrich and used as received. The molecular structures of [MMIm][MS] and [EMIm][BF4] are shown in Figure 1b and c , respectively. The MS anion was chosen so as to contain sulphonate groups to ensure chemical similarity with SS chains. The direct comparison of [EMIm][BF4] and [MMIm][MS] makes us possible to study the effect of a wide range of properties of ILs, i.e., viscosity, conductivity of pure IL, melting temperature and chemical compatibility, on ionic conductivity of polymer/IL mixtures. The molecular weight (MW), density ( d ), melting temperature ( T m ), viscosity ( η ) and conductivity ( σ ) are listed in Table 1 . Preparation of S n MB m /IL composite membranes Inhibitor-free anhydrous tetrahydrofuran (THF, ≥99.9%) was used without further purification and methanol was degassed three times before use. In the glove box, predetermined quantities of IL and S n MB m were weighed into glass vials, and approximately 5 wt% solutions were prepared using 50/50 vol% THF and methanol mixture. Solutions were stirred overnight at room temperature and approximately 200 μm thick S n MB m /IL composite membranes were prepared by solvent casting under an argon atmosphere for 2 days followed by vacuum drying at 50 °C for 10 days. Small-angle X-ray scattering The S n MB m /IL samples were laminated into an airtight sample cell consisting of an aluminium spacer, two Kapton windows, O-rings, and aluminium covers. The samples were stored with desiccant when outside the glove box to reduce the chance of water contamination. Synchrotron SAXS measurements on these samples were performed using the 4C1 SAXS beam line at the Pohang Light Source (PLS). Sample temperature was controlled within ±0.2 °C using a sample stage provided by the PLS. Samples were equilibrated for at least 15 min before measurement. The wavelength ( λ ) of the incident X-ray beam was 0.15 nm (Δ λ / λ =10 −4 ), and sample-to-detector distance of 1.5 m was used yielding scattering wave vector q ( q =4 π sin( θ /2)/ λ , where θ is the scattering angle) in the range 0.01–3.5 nm −1 . The resulting two-dimensional scattering data were averaged azimuthally to obtain intensity versus q . The scattering data were corrected for the CCD dark current and the scattering from air and Kapton windows. Transmission electron microscopy The S n MB m /IL samples prepared by the same method used to prepare the SAXS samples were cryo-microtomed at −120 °C to obtain thin sections with thicknesses in the 80–120 nm range using a Leica Ultracut UCT. The electron contrast in the samples was enhanced by exposure to ruthenium tetroxide (RuO 4 ) vapour for 50 min. Imaging of stained samples was performed with a Zeiss LIBRA 200FE microscope operating at 200 kV equipped with a cold stage (−160 °C) and an Omega energy filter. To prevent beam damage, we placed the polymer sections evacuated at 10 −5 Pa on the cold stage before they were exposed to the electron beam. Images were recorded on a Gatan 2048×2048 pixel CCD camera (Gatan Inc.). All data sets were acquired using Digital Micrograph (Gatan Inc.) software. Conductivity measurements The proton conductivities of S n MB m /IL samples were measured using AC impedance spectroscopy in glove box. The in-plane conductivity was measured using a four-electrode probe (BekkTech LLC). The probe consisted of a Teflon block, a membrane clamp, two platinum gauzes and two platinum wires. The two platinum wires were used as working and counter electrodes to apply a current to the sample membrane (2.0 cm×1.0 cm, 200 μm thick) through two platinum gauzes, and the two platinum wires 0.425 cm apart were used as reference electrodes. The normal-to-plane conductivity was measured using a home-built two-electrode cell with 1.25 cm×1.25 cm two stainless steel blocking electrodes, and 1 cm×1 cm Pt working/counter electrodes. The samples were placed in between Pt electrodes at a constant pressure of 0.8 kgf cm −2 for accurate impedance measurements. Data were collected using a 1260 Solatron impedance analyzer operating over a frequency range of 1–100,000 Hz. How to cite this article: Kim, S.Y. et al . Enhanced proton transport in nanostructured polymer electrolyte/ionic liquid membranes under water-free conditions. Nat. Commun. 1:88 doi: 10.1038/ncomms1086 (2010).